Nickel-catalyzed intermolecular oxidative Heck arylation driven by transfer hydrogenation The conventional oxidative Heck reaction between aryl boronic acids and alkenes typically involved the Pd II /Pd 0 /Pd II catalytic cycle incorporating an external oxidant and often suffered C=C bond isomerization for internal alkyl-substituted alkenes via chain-walking. Herein, we demonstrate that the regioselectivity (γ-selectivity vs. δ-selectivity) and pathway selectivity (hydroarylation vs. oxidative Heck coupling) of a directed Ni-catalyzed alkene arylation can be controlled by judicious tuning of the coordination environment around the nickel catalyst via optimization of an appropriate phosphine ligand and directing group. In this way, the Ni(0)-catalyzed oxidative Heck arylation that relies on transfer hydrogenation of an acceptor olefin is developed with excellent E / Z selectivity and regioselectivity. Mechanistic investigations suggest that the addition of the acceptor is crucial for lowering the energy for carbometalation and for enabling catalytic turnover. Transition-metal-catalyzed cross-coupling reactions involving alkenes enable conversion of abundant feedstocks to value-added products through C–C bond formation [1] , [2] , [3] , [4] , [5] , [6] , [7] , [8] , [9] , [10] , [11] , [12] , [13] , [14] , [15] , [16] . Heck-type reactions, which can be carried out both in classical polarity and oxidative modes, are the archetypal method for arene–alkene coupling. Despite significant advances during the past several decades [1] , [2] , [3] , [4] , [5] , [6] , [7] , [8] , [9] , [10] , Heck-type reactions still suffer from significant limitations, including a difficulty controlling selectivity with internal alkyl-substituted alkenes due to the lack of steric and electronic differentiation in the key migratory insertion step and issues of C=C bond isomerization due to chain-walking [17] . Additionally, though notable exceptions exist [18] , [19] , oxidative Heck reactions with arylmetal species have traditionally required use of comparatively expensive palladium catalysts with specially tailored reoxidation systems [20] , [21] , [22] , [23] , [24] , [25] , [26] . Recently, Zhou reported a highly selective Ni-catalyzed hydroarylation of styrenes and 1,3-dienes with arylboron compounds, which was proposed to proceed via oxidation addition of Ni(O) to an alcohol O–H bond to form a Ni–H species, hydrometallation across the alkene, transmetalation with the organoboron reagents, and C–C reductive elimination (Fig. 1a , path A) [27] , [28] . In 2018, we extended this strategy to hydroarylation of non-conjugated alkenes by introducing a directing group on the substrate [29] , [30] , [31] , [32] , [33] , [34] , [35] . During the course of this study, we detected byproducts arising from hydrogenolysis of the Ar–B bond, indicating that transmetalation might precede migratory insertion. In this case, a Ni(H)(Ar) intermediate would be the active form of the catalyst that engages the alkene (Fig. 1a , path B). This catalytic paradigm offers exciting possibilities for controlling regioselectivity and pathway selectivity to access different products from a common set of reagents. Fig. 1 Inspiration and motivation for the present study. a Catalytic cycle for previously reported Ni-catalyzed hydroarylation reaction. b Envisioned oxidative Heck reaction. c Relevant biologically active compounds containing γ-aryl carboxylic acid substructure Full size image We were attracted to the possibility of diverting this process to obtain non-chain-walking oxidative-Heck products by using internal alkyl-substituted alkenes and aryl boronates as the coupling partners. In the proposed cycle (Fig. 1b ), migratory insertion of the aryl group in preference to the hydride group would first take place. Subsequently, β-hydride elimination would then furnish the arylated alkene product along with a Ni(H) 2 species that would reduce a sacrificial alkene to close the catalytic cycle. If successful, this sequence of events would result in a Ni(O)-catalyzed oxidative. Heck reaction coupled to a transfer hydrogenation process [36] , [37] , [38] , [39] , [40] , [41] , [42] , [43] , [44] . We envisioned that selectivity for this pathway over other alternatives could be achieved by tuning the coordination environment around nickel with an appropriate phosphine ligand and directing group [45] , [46] , [47] , [48] , [49] , [50] , [51] , [52] . Herein we describe the realization of this goal. In particular, we report complementary transformations for both γ-selective hydroarylation and oxidative Heck coupling. These methods are efficient and scalable, providing a modular means of assembling δ-aryl olefinic acids, which are versatile building blocks for synthesizing drugs and other biologically active compounds (Fig. 1c ) [53] , [54] , [55] , [56] , [57] . 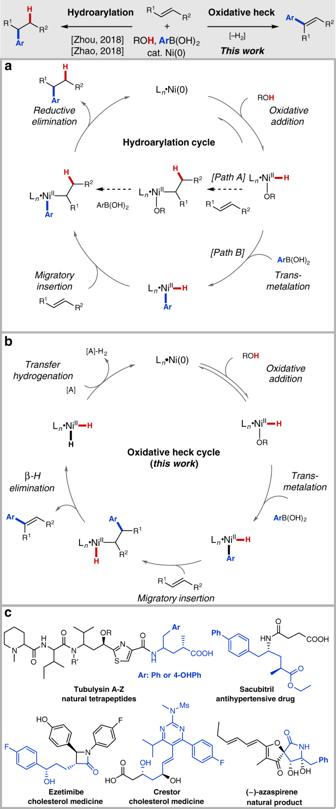Fig. 1 Inspiration and motivation for the present study.aCatalytic cycle for previously reported Ni-catalyzed hydroarylation reaction.bEnvisioned oxidative Heck reaction.cRelevant biologically active compounds containing γ-aryl carboxylic acid substructure Condition screening In a pilot experiment, 4-pentenoic acid masked with the 8-aminoquinoline (AQ) directing group ( 1a , 0.2 mmol) was subjected to our reported conditions for hydroarylation of 3-butenoic acid derivatives [29] , [58] , [59] , which gave a complicated mixture of hydoarylation and Heck-type products (Table 1 , entry 1). Next, various phosphine ligands were evaluated, and the effects were pronounced (entries 2–14). With PCy 3 or P n Bu 3 as the ligand, the δ -selective Heck-type product 5a was the major product, albeit in low yield (entries 2-3). Surprisingly, use of bulkier phosphine ligands resulted in exclusive formation of the δ-selective hydroarylation product 3a (entries 4–5). In contrast, when PMe 3 was used as the ligand, only γ-selective hydroarylation product 4a was observed in 85% yield. Notably, the γ-selectivity of this directed hydroarylation protocol is opposite to that of Loh’s Pd-catalyzed reductive Heck system, which is δ-selective for this type of substrate [60] . Using PCy 3 or P n Bu 3 as ligand, we found that adjusting the molar ratio of 1a and 2a to 1.5:1 dramatically increased the yield of oxidative Heck product 5a (entries 15–16). Notably, the reduced form of alkene 1a was detected in all the reactions, suggesting that 1a was serving as an H 2 acceptor. Based on this insight, we systematically examined various hydrogen acceptors so that alkene 1a could be used as the limiting reagent. Pleasingly, after an exhaustive screen of alkene acceptors, we identified cinnamaldehyde derivative A18 (1.0 equiv) as an efficient sacrificial alkene, and with this additive, 1 equiv 1a could be converted to 5a in 94% isolated yield. 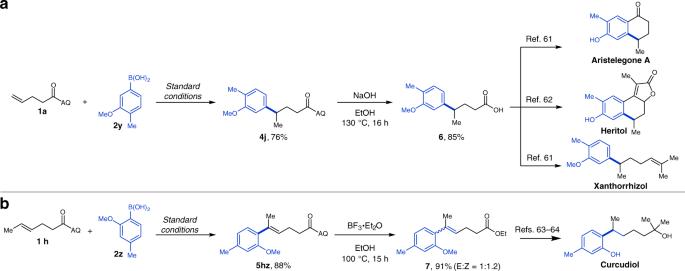Fig. 2 Synthesis of key intermediates towards natural products.aThe application of hydroarylation to approach the key intermediates in the synthesis of the natural products.bThe application of oxidative Heck coupling toward the key intermediate in the synthesis of the natural product curcudiol Table 1 Reaction optimization Full size table Substrate scope of hydroarylation Given the opposite selectivity of our Ni-catalytic system compared to Loh’s Pd-catalyzed reductive Heck system for hydroarylation of 4-pentenoic acids [60] , we next briefly probed the substrate scope of the γ-selective hydroarylation (Table 2 ). A diverse collection of arylboronic acids could be coupled to 1a , furnishing the corresponding γ-arylated products in good to excellent yields. Cyclic alkenes and δ,δ-disubstituted alkenes also underwent hydroarylation, though in these cases the reactions proceeded with δ-selectivity. Notably, these substrates are unreactive in Loh’s Pd-catalyzed system. 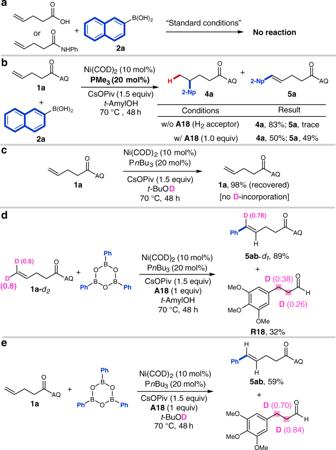Fig. 3 Experiments to elucidate Heck coupling mechanism.aControl experiments establishing the need for the AQ-directing group in both hydroarylation and Heck coupling.bThe role of the compoundA18.cThe importance of aryl boronic acid in alkene insertion.dThe reaction with δ,δ-di-deuterated alkene1a-d2.eDeuteration experiments int-BuOD Table 2 Substrate scope of hydroarylation Full size table Substrate scope of oxidative Heck reaction Next, we investigated the substrate scope and functional group tolerance of the oxidative Heck reaction with respect to the organoboron reagent using 1a as the model alkene substrate (Table 3 ). To our delight, a wide variety of para- and meta -substituted arylboronic acids with different electronic properties afforded the desired products in good to excellent yields and with high E -selectivity ( 5ae–ao ). ortho -Substituted arylboronic acids were slightly lower yielding, presumably due to steric encumbrance ( 5ac − ad ). Multi-substituted arylboronic acids ( 5ap − ar ) and heteroarylboronic acids ( 5as − av ) also provided the corresponding Heck products in high yields. Additionally, cyclic and acyclic alkenyl boronic acids were competent coupling partners, enabling access to conjugated dienoic acid derivatives ( 5aw − ax ). Importantly, this method was found to be compatible with an array of functional groups, including halo, acetyl, alkoxycarbonyl, cyano, and methoxy substituents, and could be carried out on gram scale (1.14 g of 5ab , 84%). The structure of 5a was confirmed by single-crystal X-ray diffraction. Table 3 Scope of organoboronic acids and alkenes in oxidative Heck arylation Full size table We then evaluated various γ,δ-unsaturated carboxamides (Table 3 ). Terminal alkenes bearing a single substituent at the α- or β-position reacted smoothly to afford the desired products with the complete E -selectivity ( 5ba − ea ). The β,β-disubstituted terminal alkene was also reactive, selectively furnishing desired product 5fa . In contrast, the sterically more congested α,α-disubstituted terminal alkene only gave 36% yield, even after brief optimization of the conditions ( 5ga ). ( E )-Internal alkenes bearing an alkyl group at the δ-position could also be efficiently converted into the corresponding E - configured products ( 5ha – ka ). However, aryl substitution at the δ-position led to clear attenuation of reactivity ( 5la ). Notably, when ( Z )-alkene 1i was used, the reaction stereospecifically generated ( Z )-product 5ia . In addition, the reaction was also compatible with β-substituted internal alkenes ( 5ma – na ), a γ-substituted terminal alkene ( 5oa ), and an α,δ-disubstituted alkene ( 5pa ), though in the latter two cases Z / E selectivity was low. In addition to γ,δ-unsaturated substrates, δ,ε-unsaturated AQ carboxamides were also examined. Surprisingly, with this substrate class, the connectivity of the products was the same as with the ( E )-γ,δ-unsaturated internal alkenes ( 5qa – qd ) suggesting potential alkene isomerization. A representative internal δ,ε-unsaturated alkene was unreactive in this isomerization/oxidative Heck cascade reaction. Synthetic utility To demonstrate the synthetic utility of our method, we first sought to prepare carboxylic acid 4j , a key intermediate in the synthesis of the natural products aristelegone A, heritol, and xanthorrhizol (Fig. 2 , upper panel) [61] , [62] . This intermediate has previously been synthesized through a sequence involving condensation followed by Michael addition and decarboxylation. As a second example, unsaturated carboxylic ester 7 was also prepared via δ-selective oxidative Heck arylation. Compound 7 has been employed as a key intermediate in the synthesis of the natural product curcudiol (Fig. 2 , lower panel) [63] , [64] . The literature method to access 7 involves a multi-step sequence including Grignard addition and Johnson–Claisen rearrangement. Fig. 2 Synthesis of key intermediates towards natural products. a The application of hydroarylation to approach the key intermediates in the synthesis of the natural products. b The application of oxidative Heck coupling toward the key intermediate in the synthesis of the natural product curcudiol Full size image Mechanism investigation We then carried out a series of experiments to elucidate the mechanism of the directed oxidative Heck reaction. As an initial control experiments, we first subjected two representative substrates lacking the AQ directing group, pent-4-enoic acid and N -phenylpent-4-enamide, to the standard reaction conditions using 2-naphthalenylboronic acid as the coupling partner (Fig. 3a ). In these experiments, no reaction took place, indicating that the AQ directing group on the olefin substrate is indispensable for reactivity. Next, to probe the formation of putative Ni–H species, we performed a stoichiometric reaction between t -amylOH (1.0 equiv.) and Ni(COD) 2 (1.0 equiv.) in C 6 D 6 at r.t. and analyzed the crude reaction mixture by 1 H NMR. We observed a new peak at −23.24 ppm, which is consistent with previously described Ni–H species in the literature [65] , [66] , [67] . Several additional experiments were then performed under catalytic conditions. First, we found that the addition of hydrogen acceptor A18 (1.0 equiv) under conditions that were otherwise identical to the optimal conditions for γ-selective hydroarylation resulted in a significant increase in the yield of Heck product 5a (Fig. 3b ). This result indicates that compound A18 may play a role beyond serving as a hydrogen acceptor. In particular, this additive could be bound to nickel as a ligand during the key migratory insertion event and could lower the activation energies for carbometalation compared to hydrometalation (see below). Second, we exposed alkene 1a to the reaction conditions in t- BuOD and were unable to detect deuterium incorporation (Fig. 3c ). The result is consistent with a scenario in which [Ni(H)(OR)] is inactive in alkene insertion until it undergoes transmetalation with arylboronic acid to give an active [Ni(H)(Ar)] species. Third we performed the reaction with δ,δ-di-deuterated alkene 1a - d 2 . The product, 5ab- d 1 (89% yield), contained a single deuterium atom at the δ position (Fig. 3d ). In addition, it was found that the reduced acceptor R18 was partially deuterated at both the α- and β-positions (Fig. 3d ). These results are consistent with an irreversible β-H elimination step followed by transfer hydrogenation to acceptor A18 . Last, we performed the standard reaction in t -BuOD (Fig. 3e ). There was no deuterium incorporation in the Heck product 5ab . Instead, the deuterium was transfered to the α- and β-positions of reduced acceptor R18 implying that: (1) hydrometalation of alkene 1a does not happen under the oxidative Heck reaction conditions; (2) hydrogen is transferred from t -BuOH to compound A18 as part of catalyst turnover. Fig. 3 Experiments to elucidate Heck coupling mechanism. a Control experiments establishing the need for the AQ-directing group in both hydroarylation and Heck coupling. b The role of the compound A18 . c The importance of aryl boronic acid in alkene insertion. d The reaction with δ,δ-di-deuterated alkene 1a - d 2 . e Deuteration experiments in t -BuOD Full size image To gain further insight into mechanism and the turnover-limiting step, we examined reaction kinetics at various initial concentrations of alkene 1a , aryl boronic acid 2o , acceptor A18 , and Ni(COD) 2 (See Supplementary Figs. 12 – 19 ). Based on initial rates, the reaction is first-order with respect to the Ni 0 catalyst and zeroth-order with respect to the alkene 1a , aryl boronic acid 2o , and the acceptor A18 . These results are consistent with turnover-limiting migratory insertion from a complex of the general form, [Ni(Ar)( 1a )( A18 )], as discussed more below. Additionally, we also performed a brief series of experiments to study the mechanism of the γ-selective hydroarylation (Fig. 4 ). First, we found that the alkene 1a is unreactive in the absence of arylboronic acid under the hydroarylation conditions (Fig. 4a ). However, in the presence of arylboronic acid 2a , most of the terminal alkene 1a is isomerized to internal alkene 1a’ after 5 h under the hydroarylation conditions (Fig. 4b ). In addition, we exposed alkene 1a to hydroarylation conditions in t- BuOD for 5 h. Deuterium incorporation was detected at all four positions of isomerized alkene 1a’ (Fig. 4c ). Several conclusions can be drawn from these results: (1) [Ni(H)(OR)] is unreactive in alkene insertion in the absence of arylboronic acid; (2) [Ni(H)(Ar)] species promotes isomerization of alkene 1a ; (3) internal alkene 1a’ is likely an intermediate for this γ-selective hydroarylation; and (4) isomerization of alkene 1a is reversible. Furthermore, we find that the addition of the hydrogen acceptor A18 in the hydroarylation reaction for 5 h partially inhibits the isomerization of alkene 1a and initiates the oxidative Heck arylation (Fig. 4d ). The isomerization of alkene 1a does not occur under the Heck reaction conditions (Fig. 4e ). Fig. 4 A series of experiments to study the mechanism of the γ-selective hydroarylation. a The control experiment in the absence of arylboronic acid. b The monitoring of the alkene substrate in hydroarylation for 5 h. c Deuterium incorporation into isomerized alkene. d The hydroarylation reaction in the presence of the compound A18 for 5 h. e The reaction by use of P n Bu 3 as the ligand for 5 h Full size image DFT calculations On the basis of literature reports and our own mechanistic experiments, we propose a catalytic cycle that begins with oxidation addition of Ni(O) to an alcohol O–H bond to form intermediate A . This is followed by transmetalation of the arylboronic acid, which affords the key [Ni(Ar)(H)] species (Fig. 5 ). An alternative sequence involving initial coordination of Ni(O) to the AQ group and subsequent O–H oxidation addition was also considered; however, this pathway was found to be much higher in energy (see Supplementary Fig. 21 ). 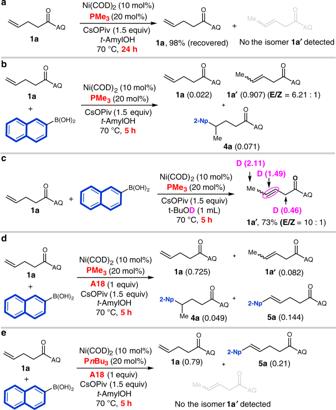Fig. 4 A series of experiments to study the mechanism of the γ-selective hydroarylation.aThe control experiment in the absence of arylboronic acid.bThe monitoring of the alkene substrate in hydroarylation for 5 h.cDeuterium incorporation into isomerized alkene.dThe hydroarylation reaction in the presence of the compoundA18for 5 h.eThe reaction by use of PnBu3as the ligand for 5 h 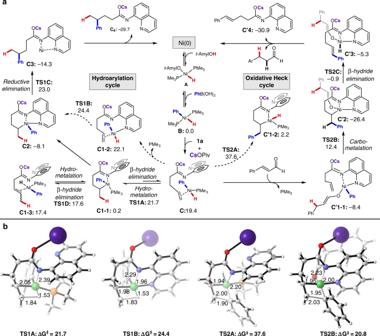Fig. 5 DFT calculations for reaction mechanism.aProposed catalytic cycle with free energies computed by DFT (kcal mol−1).bStructures of transition statesTS1A,TS1B,TS2A, andTS2B To understand the underlying origin of the divergent reactivity, DFT calculations were performed using alkene 1a and phenylboronic acid ( 2b ) as model reactants (Fig. 5 ). First, starting from [Ni(Ar)(H)] species B , ligand exchange of one PMe 3 for 1a in the presence of CsOPiv delivers complex C . Then, the reaction can proceed along two divergent pathways: Pathway I (hydroarylation; left) or Pathway II (oxidative Heck coupling; right). In Pathway I, C undergoes γ-selective hydrometalation via TS1A . The resulting six-membered nickelacycle C1-1 either directly loses a second PMe 3 ligand upon coordination of the quinoline group to form a more stable species C2 or undergoes β-hydride elimination to form C1-3 via TS1D . The other pathway to form C2 via TS1B is also possible, though it requires higher energy. Next, C2 undergoes reductive elimination via transition state TS1C to produce complex C3 . Finally, C3 releases the hydroarylated product C4 by binding a PMe 3 ligand to regenerate the Ni(O) catalyst, thereby closing the catalytic cycle. In contrast, the oxidative Heck coupling cycle proceeds in the presence of a hydrogen acceptor and involves the following steps. First, 1,4-addition of the Ni–H moiety from [Ni(Ar)(H)] species C to the hydrogen acceptor and concomitant release of PMe 3 forms intermediate C'1-1 . Subsequent carbometalation across the C=C bond via TS2B leads to formation of linear intermediate C'2 . β-Hydride elimination via TS2C results in olefinic complex C'3 , and subsequent transfer hydrogenation furnishes the product C'4 and regenerates the Ni 0 catalyst. DFT calculations indicate that: (1) the energy of direct carbometalation of C via TS2A in the absence of hydrogen acceptor is much higher than that of hydrometalation step via TS1A (37.6 vs. 21.0); and (2) the addition and coordination of hydrogen acceptor significantly lowers the energy of the carbometalation step (37.6 vs. 20.8). Therefore, the presence of a hydrogen acceptor is expected to accelerate the oxidative Heck coupling, which is consistent with the experimental results. Transition states TS2B and TS1A are close in energy (20.8 vs. 21.7), meaning that hydroarylation and Heck coupling are competitive. Fig. 5 DFT calculations for reaction mechanism. a Proposed catalytic cycle with free energies computed by DFT (kcal mol −1 ). b Structures of transition states TS1A , TS1B , TS2A , and TS2B Full size image In summary, we describe a transfer-hydrogenation-coupled oxidative Heck reaction catalyzed by a versatile Ni(O)/PR 3 /alcohol catalytic system. With the aid of a cleavable AQ directing group, a broad range of γ,δ- and δ,ε-unsaturated carboxamides, including traditionally challenging non-conjugated internal alkenes, are tolerated. The arylated alkene products are typically obtained with high E / Z selectivity and as single positional isomers. Mechanistic studies are consistent with a transfer hydrogenation process involving an active [Ni(Ar)(H)] species. The hydrogen acceptor promotes the carbometalation step and formally accepts dihydrogen from the metal. To our knowledge, intermolecular Ni(O)-catalyzed oxidative boron Heck reaction has not been reported before. General procedure for Heck arylation In an argon-filled glovebox, an oven-dried 25-mL Schlenk tube equipped with a Teflon-coated magnetic stir bar was charged successively with alkene 1 (0.2 mmol, 1.0 equiv. ), arylboronic acid 2 (0.4 mmol, 2.0 equiv. ), Ni(cod) 2 (0.02 mmol, 0.0055 g, 0.1 equiv. ), CsOPiv (0.3 mmol, 0.0702 g, 1.5 equiv. ), ( E )-3-(3,4,5-trimethoxyphenyl)acrylaldehyde A18 (0.2 mmol, 0.0444 g, 1.0 equiv. ), anhydrous t -AmylOH (1 mL), and P n Bu 3 (0.04 mmol, 0.0081 g, 0.2 equiv.). The tube was sealed with a Teflon screw cap, moved out of the glovebox, and placed on a hotplate pre-heated to 70 °C with vigorous stirring. After 48 h, the reaction mixture was cooled to room temperature and diluted with EtOAc. The organic layer was washed with brine solution and was then dried over anhydrous MgSO 4 . The reaction mixture was filtered through a short pad of Celite, and the solvent was evaporated under vacuum to give the crude product. The resulting residue was purified by silica gel flash column chromatography (hexane/EtOAc = 10/1) to afford the corresponding product. For details of the synthetic procedures and NMR spectra of these compounds in this manuscript see Supplementary information .